In-vitroderived germinal centre B cells differentially generate memory B or plasma cellsin vivo In response to T cell-dependent antigens, B cells proliferate extensively to form germinal centres (GC), and then differentiate into memory B (B mem ) cells or long-lived plasma cells (LLPCs) by largely unknown mechanisms. Here we show a new culture system in which mouse naïve B cells undergo massive expansion and isotype switching, and generate GC-phenotype B (iGB) cells. The iGB cells expressing IgG1 or IgM/D, but not IgE, differentiate into B mem cells in vivo after adoptive transfer and can elicit rapid immune responses with the help of cognate T cells. Secondary culture with IL-21 maintains the proliferation of the iGB cells, while shifting their in vivo developmental fate from B mem cells to LLPCs, an outcome that can be reversed by withdrawal of IL-21 in tertiary cultures. Thus, this system enables in vitro manipulation of B-cell fate, into either B mem cells or LLPCs, and will facilitate dissection of GC-B cell differentiation programs. Memory B (B mem ) cells and long-lived plasma cells (LLPCs) are the effectors of immunological memory, a hallmark of adoptive immunity, and are crucial to protect the host against recurrent infection. These cells are typically generated in germinal centres (GCs) formed in the peripheral lymphoid tissues during the T-cell-dependent (TD) immune response. In the TD response, antigen (Ag)-specific B cells present the Ag to primed cognate Th cells in the lymphoid follicles and clonally proliferate on receiving signals such as CD40-ligand (CD40L) and IL-4 from the Th cells. Some of the responding B cells leave the follicles and form extrafollicular foci of plasmablasts, which differentiate into short-lived plasma cells that survive for only a few days. Other B cells proliferate extensively in the follicles with the help of follicular helper T (Tfh) cells to form GCs, in which B cells undergo isotype switching, typically to IgG subclasses, and somatic hypermutation (SHM) of Ig genes to diversify the affinity of their B-cell receptor (BCR) for Ag [1] . Finally, GC B cells expressing a high-affinity IgG BCR are selected and differentiate into B mem cells and LLPCs by largely unknown mechanisms [2] , [3] , [4] . Some of IgG + GC B cells further switch their BCR to IgE, but the IgE + GC B cells are localized outside GCs and rapidly differentiate into plasma cells [5] . In the TD response, the CD40–CD40 ligand (CD40L) interaction is required for Th-mediated B-cell activation and thus for GC formation, and for generation of B mem cells [6] , [7] , [8] . In addition, IL-21 signalling is required for IgG1 production, efficient GC formation, affinity maturation and LLPC formation, but not for B mem cell development in mice [9] , [10] , [11] , [12] . IL-21 induces class switch recombination (CSR) to IgG [13] and Blimp1 expression in B cells through transcriptional activation of the Blimp1-enoding Prdm1 gene via cooperation of Irf4 and Stat3 (refs 14 , 15 ), and thus PC differentiation [14] , [16] , [17] , [18] . IL-21 was also reported to be required for generation of Tfh cells, which themselves produce IL-21 (refs 19 , 20 ), but this idea has recently been questioned [9] , [10] , [11] . Numerous studies have shown that the transcription factor Bcl-6 is essential for the differentiation of Tfh cells [21] and GC B cells, affinity maturation and LLPC formation, but not for B mem cell development [22] . Together, these data suggest a model in which GC B-cell differentiation, which is dependent on IL-21 signalling and Bcl-6, is a necessary prerequisite for production of the high-affinity B mem cells and LLPCs, but is not essential for B mem cell generation per se . Thus, signalling and transcriptional programs that determine B mem cell fate are still unknown. Similarly, it remains unclear what determines lineage choice by the affinity-selected GC B cells to become LLPCs, although transcriptional regulators such as Blimp-1 and Irf4 are known to be essential for overall plasma cell differentiation [23] , [24] . A study to elucidate molecular mechanisms for the fate decision of GC B cells in mice is challenging, because the numbers of B mem cells and LLPCs, and presumably their precursors in GCs, are too few to be experimentally manipulated ex vivo . Moreover, there is no definitive marker for B mem cells in mice. B7.1 (CD80) [25] and CD38 (ref. 26 ) are useful but not B mem -specific markers. Thus, B mem cells have been identified as B cells expressing Ag-specific IgG in immunized mice, but B mem cells bearing unswitched BCR (IgM + IgD + ) have also been recognized [27] , [28] , [29] . Functionally, B mem cells can be defined as long-lived Ag-experienced B cells that rapidly produce Ab in response to re-challenge with soluble, adjuvant-free Ags after being transferred into recipient mice together with cognate Th cells [30] . This assay should be potentially useful to identify factors that affect development, longevity, in situ localization, Ag responsiveness and so on of B mem cells, but their paucity and in vitro fragility have limited these applications, except for using specific mutant mouse strains [27] , [31] , [32] . In vitro culture systems that allow long-term proliferation of primary T cells and their differentiation towards specific T cell subsets, for example, Th1, Th2, Th17 or Tregs, have been established and broadly used to study molecular mechanisms for T-cell differentiation. A culture system for human B cells, in which tonsil GC B cells can differentiate to either the PC or B mem phenotype, was previously reported [33] , [34] , [35] , although functional studies of the human B mem cells remain extremely difficult. Mouse B cells are known to proliferate, undergo class switching and differentiate into plasma cells in response to stimulation with anti-Ig Ab, LPS, anti-CD40 Ab, and/or cytokines, such as IL-4, in vitro , but the resulting cell growth is transient and the cells die within days. Thus, there has been no practical in vitro system to propagate B cells and then control their differentiation towards B mem cell or LLPC lineages. Here we describe a new in vitro culture system in which naïve murine B cells proliferate enormously, exhibit a GC B cell phenotype, and develop into either B mem cells or LLPCs in vivo after adoptive transfer. With this system, we have clearly demonstrated a role for IL-21 in determination of the GC B cell fate, the reversible suppression of B mem cell commitment. A new culture system to propagate GC phenotype B cells To propagate B cells in vitro , we generated three feeder cell lines: BALB/c 3T3 fibroblasts stably transfected with both CD40L and BAFF (40LB) ( Fig. 1a ) or individually with either CD40L (3T3/40L) or BAFF (3T3/BAFF). We cultured naïve splenic B cells on these feeder cells in the presence of IL-4. The B cells proliferated on 40LB cells and the live cell number increased, resulting in a 180-fold expansion after 6 days ( Fig. 1b ), whereas there was minimal proliferation on 3T3/40L, 3T3/BAFF or 3T3 cells. On 3T3/BAFF cells, the B cell number increased less than tenfold by co-stimulation with anti-CD40 Ab and IL-4, and the expansion was even less with IL-4 and LPS ( Fig. 1b ). These differences in expansion were due partly to differences in DNA synthesis as demonstrated by BrdU incorporation ( Fig. 1c ). CFSE-labelling analysis also revealed that the all B cells replicated more rapidly on 40LB cells with IL-4 than without, whereas B cells on 3T3/BAFF with anti-CD40 and IL-4 replicated more slowly and heterogeneously ( Fig. 1d ). These data indicate that co-expression of membrane-bound CD40L and BAFF is required for the feeder cells to support optimum proliferation of B cells. 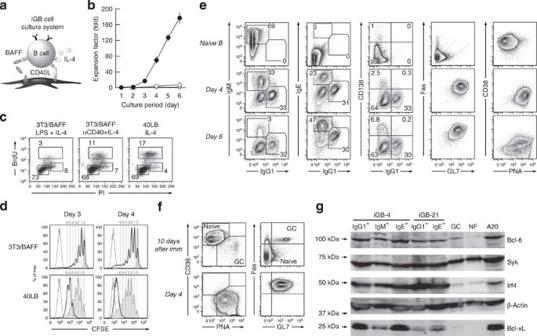Figure 1:In vitroinduction and massive expansion of phenotypically GC B cells from naïve B cells. (a) Schematic representation of the iGB cell culture system. (b) Cumulative fold increase in the number of live B cells cultured on 40LB with IL-4 (closed circles), on 3T3/BAFF with anti-CD40 Ab (1 μg ml−1) plus IL-4 (open circles), or on 3T3/BAFF with LPS (10 μg ml−1) plus IL-4 (shaded circles). Shown are mean values with s.d. at the indicated time points from three independent experiments, each done singly from an individual mouse. (c) B cells were cultured as in (b) for 3 days and pulsed with BrdU for the last 1 h. The cells were stained with anti-BrdU Ab and propidium iodide and analysed by flow cytometry. Numbers indicate the percentages of the cells in the G1 (lower left window), S (upper window), and G2-M (lower right window) phases of cell cycle. The data shown are representative of two independent experiments. (d) CFSE-labelled splenic naïve B cells were cultured for 3 or 4 days on 3T3/BAFF with anti-CD40 Ab (1 μg ml−1) plus IL-4 (thick line) or without (shaded) ('3T3/BAFF'), or on 40LB with IL-4 (thick line) or without (shaded) ('40LB'), and then analysed by flow cytometry. Unlabelled B cells cultured on 40LB with IL-4 served as negative controls (thin line). Theoretical cell division numbers are noted on top of each histogram. The data shown are representative of three independent experiments. (e) Flow cytometric analysis for the indicated markers of iGB cells cultured with IL-4 for 4 or 6 days, or of splenic naïve B cells from a C57BL/6 mouse. Expression of Fas, GL7, CD38, and PNA ligand was analysed for CD138−gated cells. Numbers indicate the percentages of cells in the indicated quadrants or windows. The data shown are representative of numerous independent experiments. (f) Flow cytometric analysis of iGB cells cultured with IL-4 for 4 days (day 4), and of pooled splenic B cells from three mice that had been immunized with 100 μg of NP-CGG/alum 10 days before (10 days after imm). Expression of CD38, PNA ligand, Fas and GL7 on CD19+CD138–gated cells is shown. (g) Western blot analysis was performed using the following cells purified by the FACSAria II cell sorter: IgG1+, IgM+or IgE+, CD138−populations from iGB cells 4 days after primary culture with IL-4 (iGB-4), and IgG1+or IgE+, CD138−populations from those after the subsequent culture for 2 more days with IL-21 (iGB-21), splenic GC B cells (GC: GL7+, Fas+, CD19+, CD138−) from 20 C57BL/6 mice immunized with BSA/CFA 2 weeks earlier, splenic naïve follicular B cells (NF: CD21+, CD23high, CD19+, CD43−) from unimmunized C57BL/6 mice. IgG+mouse B-lymphoma cell line A20 was used as a control. All samples consist of 2×106cells per lane, except the IgM+iGB-4 ells (1×106cells). The blot was probed with antibodies against indicated proteins. Figure 1: In vitro induction and massive expansion of phenotypically GC B cells from naïve B cells. ( a ) Schematic representation of the iGB cell culture system. ( b ) Cumulative fold increase in the number of live B cells cultured on 40LB with IL-4 (closed circles), on 3T3/BAFF with anti-CD40 Ab (1 μg ml −1 ) plus IL-4 (open circles), or on 3T3/BAFF with LPS (10 μg ml −1 ) plus IL-4 (shaded circles). Shown are mean values with s.d. at the indicated time points from three independent experiments, each done singly from an individual mouse. ( c ) B cells were cultured as in ( b ) for 3 days and pulsed with BrdU for the last 1 h. The cells were stained with anti-BrdU Ab and propidium iodide and analysed by flow cytometry. Numbers indicate the percentages of the cells in the G1 (lower left window), S (upper window), and G2-M (lower right window) phases of cell cycle. The data shown are representative of two independent experiments. ( d ) CFSE-labelled splenic naïve B cells were cultured for 3 or 4 days on 3T3/BAFF with anti-CD40 Ab (1 μg ml −1 ) plus IL-4 (thick line) or without (shaded) ('3T3/BAFF'), or on 40LB with IL-4 (thick line) or without (shaded) ('40LB'), and then analysed by flow cytometry. Unlabelled B cells cultured on 40LB with IL-4 served as negative controls (thin line). Theoretical cell division numbers are noted on top of each histogram. The data shown are representative of three independent experiments. ( e ) Flow cytometric analysis for the indicated markers of iGB cells cultured with IL-4 for 4 or 6 days, or of splenic naïve B cells from a C57BL/6 mouse. Expression of Fas, GL7, CD38, and PNA ligand was analysed for CD138 − gated cells. Numbers indicate the percentages of cells in the indicated quadrants or windows. The data shown are representative of numerous independent experiments. ( f ) Flow cytometric analysis of iGB cells cultured with IL-4 for 4 days (day 4), and of pooled splenic B cells from three mice that had been immunized with 100 μg of NP-CGG/alum 10 days before (10 days after imm). Expression of CD38, PNA ligand, Fas and GL7 on CD19 + CD138 – gated cells is shown. ( g ) Western blot analysis was performed using the following cells purified by the FACSAria II cell sorter: IgG1 + , IgM + or IgE + , CD138 − populations from iGB cells 4 days after primary culture with IL-4 (iGB-4), and IgG1 + or IgE + , CD138 − populations from those after the subsequent culture for 2 more days with IL-21 (iGB-21), splenic GC B cells (GC: GL7 + , Fas + , CD19 + , CD138 − ) from 20 C57BL/6 mice immunized with BSA/CFA 2 weeks earlier, splenic naïve follicular B cells (NF: CD21 + , CD23 high , CD19 + , CD43 − ) from unimmunized C57BL/6 mice. IgG + mouse B-lymphoma cell line A20 was used as a control. All samples consist of 2×10 6 cells per lane, except the IgM + iGB-4 ells (1×10 6 cells). The blot was probed with antibodies against indicated proteins. Full size image We next analysed the phenotype of the B cells growing on 40LB by flow cytometry. As expected, IL-4 induced BCR class switching from IgM to IgG1 and IgE, generating discrete populations of IgG1 + and IgE + cells by day 4 ( Fig. 1e ). The IgE + cell population further increased in frequency with time, whereas the IgG1 − IgE − cell population, consisting mostly of IgM + IgD + cells, decreased. A small fraction of the IgG1 − cells (mostly IgE + ) were CD138 + and these increased in frequency with time. All but the CD138 + cells exhibited a cell-surface phenotype typical of GC B cells: GL7 + Fas + CD38 low and PNA + ( Fig. 1e ), comparable to ex vivo GC B cells in the spleen of immunized mice ( Fig. 1f ). The expression of CCR7 on the iGB cells was as similar to naïve follicular B cells ( Supplementary Fig. S1 ), as reported for mouse GC B [36] , and unlike the high CCR7 levels seen on activated B cells [37] . Thus, we call these B cells propagated on 40LB cells in-vitro -induced GC B (iGB) cells. The IgG1 + , IgE + or IgM + , CD138 − populations of iGB cells on day 4 expressed abundant Bcl-6 and Bcl-xL proteins, at a level even higher than the ex vivo GC B cells ( Fig. 1g ). Both proteins have recently been shown to be significantly higher in mouse GC B cells than in follicular B cells [38] , showing that iGB cells share some molecular features with GC B cells. Generation of B mem cells from iGB cells in vivo B mem cells typically develop from GC B cells, but B mem cells with unmutated Igs can develop in mice lacking discernable GCs [27] . Therefore, we assessed whether the iGB cells contain B mem cell precursors. iGB cells expressing an allelic marker (Ly5.1 + ) were transferred intravenous (i.v.) into irradiated C57BL/6 (Ly5.2 + ) mice. Eight weeks later, a significant population of donor-derived B cells (Ly5.1 + , CD19 + ) was detected in the spleen ( Fig. 2a ). In contrast to the recipient B cells, which were uniformly IgM/D + , about two-thirds of these cells were IgG1 +, and the rest were IgM + IgD + (IgM/D + ). Notably, donor-derived IgE + cells were never found in repeated experiments. Compared with recipient-derived naïve B cells, donor-derived IgG1 + and IgM/D + B cells were larger and expressed higher levels of B7.1, CD21, CD19 and MHC class-II. Although the iGB cells expressed high levels of the GC B-cell markers Fas and GL7, after transfer, they expressed only moderate levels of Fas and were GL7 negative ( Fig. 2b,c ). Additionally, they were CD38 high and CD62L int , markers that are both low on GC as well as iGB cells. The donor-derived cells had lower CD23 levels than naïve B cells, and little of the CD138 and CD43 PC markers ( Fig. 2b ). These results indicate that a significant number of the transferred iGB cells survived for long periods in the spleen of the recipient mice and acquired the phenotype of B mem cells, which were designated induced memory B (iMB) cells. 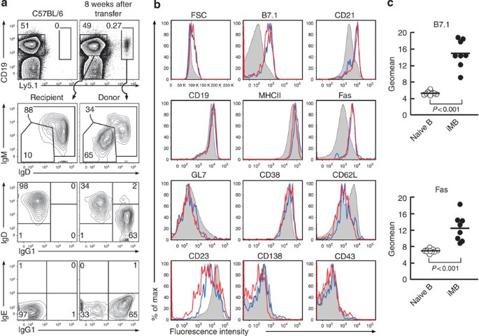Figure 2: iGB cells differentiate into cells with a Bmemphenotype in recipient mice. (a) Day 4 iGB cells derived from C57BL/6 Ly5.1+congenic mice (2×107) were purified and transferred i.v. into γ-irradiated (6.5 Gy) C57BL/6 mice (Ly5.2+). Eight weeks later, pooled spleens of four recipients and a spleen of an untreated C57BL/6 mouse were stained with the indicated antibodies and analysed by flow cytometry. Ly5.1+CD19+donor and Ly5.1−CD19+recipient B cells were gated as indicated and analysed for their BCR isotypes. (b) Expression of the indicated markers on the donor IgG1+(Ly5.1+CD19+IgD−: red line) or IgM/D+(Ly5.1+CD19+IgD+: blue line) iMB cells and the recipient naïve B cells (Ly5.1−CD19+IgD+: shaded) shown in (a) were analysed. Anti-mouse IgG1 Ab was not used because it often cross-reacts with rat antibodies. The data shown are representative of three independent experiments performed with three to four mice per group. (c) Expression levels of B7.1 and Fas on Ly5.1+iMB cells (closed circles;n=8) or Ly5.1−naïve B cells from the recipient and two normal C57BL/6 mice (open circles;n=10). Plotted are geometric means (geomean) of the fluorescence intensity of the cells from individual mice with the average value of each group of mice indicated by a horizontal line. Figure 2: iGB cells differentiate into cells with a B mem phenotype in recipient mice. ( a ) Day 4 iGB cells derived from C57BL/6 Ly5.1 + congenic mice (2×10 7 ) were purified and transferred i.v. into γ-irradiated (6.5 Gy) C57BL/6 mice (Ly5.2 + ). Eight weeks later, pooled spleens of four recipients and a spleen of an untreated C57BL/6 mouse were stained with the indicated antibodies and analysed by flow cytometry. Ly5.1 + CD19 + donor and Ly5.1 − CD19 + recipient B cells were gated as indicated and analysed for their BCR isotypes. ( b ) Expression of the indicated markers on the donor IgG1 + (Ly5.1 + CD19 + IgD − : red line) or IgM/D + (Ly5.1 + CD19 + IgD + : blue line) iMB cells and the recipient naïve B cells (Ly5.1 − CD19 + IgD + : shaded) shown in ( a ) were analysed. Anti-mouse IgG1 Ab was not used because it often cross-reacts with rat antibodies. The data shown are representative of three independent experiments performed with three to four mice per group. ( c ) Expression levels of B7.1 and Fas on Ly5.1 + iMB cells (closed circles; n =8) or Ly5.1 − naïve B cells from the recipient and two normal C57BL/6 mice (open circles; n =10). Plotted are geometric means (geomean) of the fluorescence intensity of the cells from individual mice with the average value of each group of mice indicated by a horizontal line. Full size image Generation of iMB cells is independent of antigenic stimulation B mem cells are maintained with no or very slow cycling [39] , so we asked whether the iMB cells are cycling in vivo . BrdU-pulsed iGB cells were transferred into irradiated mice and their kinetics were analysed. At the time of transfer, 73% of IgG1 + cells were BrdU + and after two weeks ∼ 30% of the cells were BrdU + , a percentage that remained largely unchanged even at 8 weeks after the transfer ( Fig. 3a,b ). These data indicate that the iMB cells became quiescent during the 6 weeks after the point of 2 weeks post-transfer, a time by which none of the donor B cells had the GC phenotype but exhibited the B mem phenotype. These results indicate that, after the B mem phenotype is established, IgG1 + iMB cells are maintained with very little, if any, cycling in vivo . Very similar results were observed with IgM/D + iMB cells ( Supplementary Fig. S2 ). 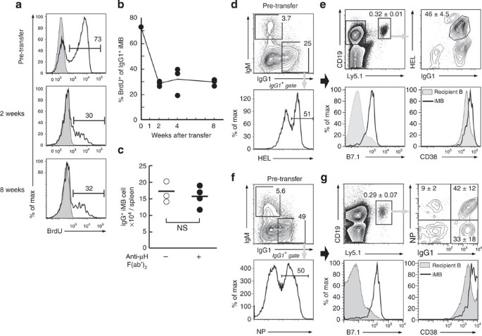Figure 3: Generation and maintenance of iMB cells are independent of antigenic stimulation. (a,b)In vivoBrdU-pulse chase analysis of iMB cells. Ly5.1+iGB cells were pulsed with BrdU or not for the last 7 h of a 4-day culture and then transferred into irradiated (6.5 Gy) C57BL/6 mice. BrdU content was analysed by flow cytometry in the IgG1+pre-transfer iGB cells (n=1) and IgG1+Ly5.1+CD19+donor iMB cells in the spleens of the recipient mice 2, 4, or 8 weeks after transfer (n=3 for each time point). (a) Representative data with numbers indicating percentages of BrdU-containing pre-transfer and iMB cells. Unpulsed iGB and iMB cells are shown as controls (shaded). (b) Kinetics of the percentage of BrdU+iMB cells in individual recipients. The value of pre-transfer cells is plotted at 0-week. Data shown are representative of two independent experiments. (c) The effect of initial BCR stimulationin vitroon iMB generationin vivo. Mice had received Ly5.1+iGB cells cultured with (closed circles:n=4) or without (open circles:n=3) extra anti-μH F(ab′)2(1 μg ml−1) 62 days before. Absolute numbers, with an average in each group (horizontal bars), of IgG1+CD19+Ly5.1+iMB cells in each spleen of individual recipient mice are plotted. The cell number is estimated on the basis of the cell frequency determined by flow cytometry and total cell number. n.s.: not significant. Similarly, no effect of BCR stimulation was observed in the recipients 20 days after transfer in an independent experiment. (d–g) Day 4 iGB cells derived from total splenic B cells from Hy10 Ly5.1+mice (d) or those enriched for NP+cells from B1-8 ki Ly5.1+mice (f) were transferred into irradiated C57BL/6 mice. The frequency of IgM+and IgG1+cells (d,f), and of IgG1+cells binding to HEL (d) or NP (f) antigens in the pre-transfer iGB cells are shown. For unknown reasons, the iGB cells with a knock-in IgH gene tend to undergo isotype switching more rapidly and to express lower BCR levels than wild-type iGB cells. (e) The frequencies of Ly5.1+CD19+iMB cells in the pooled spleen cells from four recipient mice 37 days after transfer with the cells shown in (d), and profiles of these iMB cells illustrating antigen-binding and IgG1 expression, B7.1 expression, and CD38 expression, are shown. (g) The frequency of iMB cells in the pooled spleen cells from four recipient mice 91 days after transfer with the cells shown in (f), and the same profiles as above, are shown. Data are representative of three or more experiments each performed with two-to-five recipient mice. Figure 3: Generation and maintenance of iMB cells are independent of antigenic stimulation. ( a , b ) In vivo BrdU-pulse chase analysis of iMB cells. Ly5.1 + iGB cells were pulsed with BrdU or not for the last 7 h of a 4-day culture and then transferred into irradiated (6.5 Gy) C57BL/6 mice. BrdU content was analysed by flow cytometry in the IgG1 + pre-transfer iGB cells ( n =1) and IgG1 + Ly5.1 + CD19 + donor iMB cells in the spleens of the recipient mice 2, 4, or 8 weeks after transfer ( n =3 for each time point). ( a ) Representative data with numbers indicating percentages of BrdU-containing pre-transfer and iMB cells. Unpulsed iGB and iMB cells are shown as controls (shaded). ( b ) Kinetics of the percentage of BrdU + iMB cells in individual recipients. The value of pre-transfer cells is plotted at 0-week. Data shown are representative of two independent experiments. ( c ) The effect of initial BCR stimulation in vitro on iMB generation in vivo . Mice had received Ly5.1 + iGB cells cultured with (closed circles: n =4) or without (open circles: n =3) extra anti-μH F(ab′) 2 (1 μg ml −1 ) 62 days before. Absolute numbers, with an average in each group (horizontal bars), of IgG1 + CD19 + Ly5.1 + iMB cells in each spleen of individual recipient mice are plotted. The cell number is estimated on the basis of the cell frequency determined by flow cytometry and total cell number. n.s. : not significant. Similarly, no effect of BCR stimulation was observed in the recipients 20 days after transfer in an independent experiment. ( d – g ) Day 4 iGB cells derived from total splenic B cells from Hy10 Ly5.1 + mice ( d ) or those enriched for NP + cells from B1-8 ki Ly5.1 + mice ( f ) were transferred into irradiated C57BL/6 mice. The frequency of IgM + and IgG1 + cells ( d , f ), and of IgG1 + cells binding to HEL ( d ) or NP ( f ) antigens in the pre-transfer iGB cells are shown. For unknown reasons, the iGB cells with a knock-in IgH gene tend to undergo isotype switching more rapidly and to express lower BCR levels than wild-type iGB cells. ( e ) The frequencies of Ly5.1 + CD19 + iMB cells in the pooled spleen cells from four recipient mice 37 days after transfer with the cells shown in ( d ), and profiles of these iMB cells illustrating antigen-binding and IgG1 expression, B7.1 expression, and CD38 expression, are shown. ( g ) The frequency of iMB cells in the pooled spleen cells from four recipient mice 91 days after transfer with the cells shown in ( f ), and the same profiles as above, are shown. Data are representative of three or more experiments each performed with two-to-five recipient mice. Full size image We examined whether BCR signalling is involved in the generation of iMB cells in vivo and found that stimulation of iGB cells with anti-μH F(ab′) 2 Ab during the culture period did not affect the number of the resultant IgG1 + or IgM/D + iMB cells in the recipient spleens ( Fig. 3c ; Supplementary Fig. S2 ). We next generated iGB cells from two mouse lines, each expressing knock-in/transgenic BCR specific for a known external antigen: Hy10 (refs 40 , 41 ), which is specific for hen egg lysozyme (HEL), and B1-8 ki [42] , which is specific for (4-hydroxy-3-nitrophenyl) acetyl (NP) when co-expressing λ L chains. The iGB cells derived from these mice, about half of which were Ag specific, ( Fig. 3d,f ), gave rise to iMB cells in the recipients at a frequency similar to the non-transgenic B cells, and, moreover, these iMB cells could persist as long as 3 months without antigen. The iMB cells in both cases exhibited a B mem phenotype (B7.1 + and CD38 high ) and maintained the same proportion of IgG1 + antigen-binding B cells as in the pre-transfer cells ( Fig. 3e,g ). These data indicate that antigenic stimulation is not required for generation of iMB cells. iMB cells function as B mem cells To investigate whether iMB cells rapidly respond to T-dependent (TD) adjuvant-free antigen similarly to physiological B mem cells, mice containing Hy10-derived iMB cells, generated as in Figure 3e , were injected with splenocytes containing memory T cells primed with ovalbumin (OVA) and then immunized i.v. with a soluble OVA-HEL conjugate. Five days later, spleens of the recipient mice were analysed by flow cytometry ( Fig. 4a ). The unimmunized control mice contained a single population of iMB cells that had high levels of HEL binding (HEL high ), whereas the immunized mice contained another population of donor-derived cells that bound less HEL (HEL low ). HEL high iMB cells in both mice exhibited the B mem phenotype whereas HEL low cells in the immunized mice were larger and mostly exhibited a plasmablast phenotype: CD138 + , CD43 + , CD19 low , surface IgG1 low , and CD38 low . Using immunofluorescence microscopy, we showed that, in unimmunized mice, HEL + iMB cells were localized in the perifollicular regions and mostly scattered along the MAdCAM-1 + marginal sinus ( Fig. 4b–d ). In the immunized mice, most of the HEL + IgG1 + cells were localized in the extrafollicular regions, in the red pulp or at the junction of the T-cell zone and the red pulp ( Fig. 4e–g ). The HEL + iMB cells did not form GCs in the follicles, as has also been reported for bona fide B mem cells [43] . 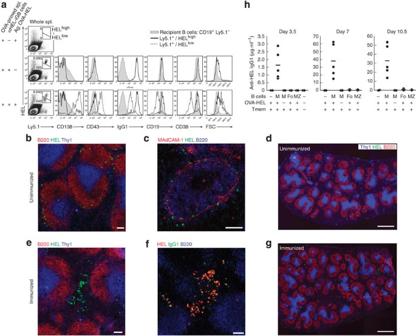Figure 4: iMB cells rapidly differentiate into plasma cellsin vivoon immunization. (a) Control C57BL/6 mice (αHEL-iGB cells: −) or mice that received Hy10 Ly5.1+iGB cells 50 days before (αHEL-iGB cells: +) were injected i.v. with 2×107pooled splenocytes from mice primed with OVA with CFA 2 months before, and immunized i.v. with OVA-HEL (20 μg) in PBS (Ag:OVA-HEL: +) or not (Ag:OVA-HEL: −) 12 h later. Five days after immunization, spleen cells were analysed by flow cytometry. Each histogram shows the staining profile of the indicated marker in Ly5.1+HELhighor HELlowdonor B cells and CD19+Ly5.1−recipient B cells defined in the dot plots. (b–g) Photomicrographs of sections of the same spleens of the mice receiving iGB cells in (a), unimmunized (b–d) or immunized (e–g). Sections were stained with anti-B220 (red), HEL (green), and anti-Thy1 (blue) (b,d,e,g); anti-MAdCAM-1 (red), HEL (green), and anti-B220 (blue) (c); or HEL (red), anti-IgG1 (green), and anti-B220 (blue) (f). Data are representative of three independent experiments. Magnification is ×20 (b,c,e,f) or ×4 (d,g). Bars: 100 μm (b,c,e,f) or 1 mm (d,g). (d,g) show low power views of the images in (b) and (e), respectively. (h) Splenocytes (2×107) from OVA-primed mice (Tmem) were transferred i.v. into non-irradiated C57BL/6 mice with the HEL+iMB cell-containing splenic B cells shown inFigure 3d(M) (n=5), with sorted HEL+follicular B cells (Fo) (n=2) or MZ B cells (MZ) (n=2) from naïve Hy10 mice, or without B-cells (−) (n=2). All donor B cells contained 1.2×105HEL+B cells. After i.v. immunization with (+) or without (−) 20 μg OVA-HEL, serum titres of anti-HEL IgG1 in individual mice were determined on the indicated days. Horizontal bars indicate the average value in each group. Data shown are representative of three independent experiments performed with two-to-five mice per group. Figure 4: iMB cells rapidly differentiate into plasma cells in vivo on immunization. ( a ) Control C57BL/6 mice (αHEL-iGB cells: −) or mice that received Hy10 Ly5.1 + iGB cells 50 days before (αHEL-iGB cells: +) were injected i.v. with 2×10 7 pooled splenocytes from mice primed with OVA with CFA 2 months before, and immunized i.v. with OVA-HEL (20 μg) in PBS (Ag:OVA-HEL: +) or not (Ag:OVA-HEL: −) 12 h later. Five days after immunization, spleen cells were analysed by flow cytometry. Each histogram shows the staining profile of the indicated marker in Ly5.1 + HEL high or HEL low donor B cells and CD19 + Ly5.1 − recipient B cells defined in the dot plots. ( b – g ) Photomicrographs of sections of the same spleens of the mice receiving iGB cells in ( a ), unimmunized ( b – d ) or immunized ( e – g ). Sections were stained with anti-B220 (red), HEL (green), and anti-Thy1 (blue) ( b , d , e , g ); anti-MAdCAM-1 (red), HEL (green), and anti-B220 (blue) ( c ); or HEL (red), anti-IgG1 (green), and anti-B220 (blue) ( f ). Data are representative of three independent experiments. Magnification is ×20 ( b , c , e , f ) or ×4 ( d , g ). Bars: 100 μm ( b , c , e , f ) or 1 mm ( d , g ). ( d , g ) show low power views of the images in ( b ) and ( e ), respectively. ( h ) Splenocytes (2×10 7 ) from OVA-primed mice (T mem ) were transferred i.v. into non-irradiated C57BL/6 mice with the HEL + iMB cell-containing splenic B cells shown in Figure 3d (M) ( n =5), with sorted HEL + follicular B cells (Fo) ( n =2) or MZ B cells (MZ) ( n =2) from naïve Hy10 mice, or without B-cells (−) ( n =2). All donor B cells contained 1.2×10 5 HEL + B cells. After i.v. immunization with (+) or without (−) 20 μg OVA-HEL, serum titres of anti-HEL IgG1 in individual mice were determined on the indicated days. Horizontal bars indicate the average value in each group. Data shown are representative of three independent experiments performed with two-to-five mice per group. Full size image To examine Ab production by iMB cells, splenic B cells containing HEL + iMB cells shown in Figure 3e or naïve follicular or marginal zone (MZ) B cells from Hy10 mice were co-transferred with splenocytes from OVA-primed mice into secondary recipient mice. On immunization i.v. with soluble OVA-HEL, the mice that received HEL + iMB cells produced anti-HEL IgG1 Ab, which was detectable as early as day 3.5 and peaked by day 7 after immunization, but mice that received naïve follicular or MZ B cells or no HEL + B cells did not respond ( Fig. 4h ). Similar results were observed in the model of NP + iMB cells and carrier-primed CD4 + T cells ( Fig. 3g ; Supplementary Fig. S3 ). When Hy10-derived IgG1 + and IgM/D + iMB cells were separately transferred into mice with OVA-primed T cells, both types of iMB cells responded to immunization with soluble OVA-HEL, as shown by expansion, differentiation into CD138 + plasmablasts, and production of anti-HEL IgG1 at equivalent levels ( Supplementary Fig. S4 ). These results indicate that, in the presence of memory T H cells, iMB cells are able to differentiate rapidly into plasmablasts and begin to produce Ab after immunization with soluble, adjuvant-free TD antigen. Taken together with the other iMB cell features described above, we conclude that iMB cells are phenotypically and functionally equivalent to physiological B mem cells. IL-21 boosts proliferation of IL-4-induced iGB cells IL-21 is required for maximal expansion of GC B cells [9] , [10] , [11] , [12] , and facilitates proliferation of BCR-/CD40-stimulated B cells [14] , [44] . Primary culture with IL-21 on 40LB feeder cells for 4 days resulted in 25-fold less proliferation of B cells than in the cultures with IL-4, with less frequent or little switching to IgG1 and IgE, respectively. Despite the known synergistic effect of IL-4 and IL-21 for Ig production in vivo [12] , synergy in proliferation was not evident in the primary cultures ( Supplementary Fig. S5 ). Next, iGB cells were first cultured with IL-4 and then subsequently cultured for 2 days either with IL-21 or IL-4 ( Fig. 5a ). 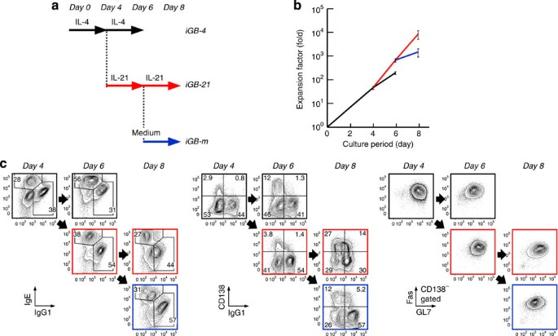Figure 5: IL-21 accelerates proliferation of iGB cells and partial differentiation of IgG1+iGB cells into plasmablasts. (a) Schematic diagram of the different iGB cell cultures performed in (b,c).In vitrogenerated iGB cells were successively cultured on 40LB cells with IL-4 (iGB-4; black), or with IL-21 replacing IL-4 on day 4 (iGB-21; red). Additionally, the iGB-21 cells were deprived of IL-21 on day 6 and successively cultured on 40LB without added cytokines (iGB-m; blue). (b) Cumulative fold increase on day 4, 6, and 8, of B cells cultured as described in (a) was estimated from three independent experiments and represented as inFigure 1b. Colours of the lines indicate the culture conditions described in (a). (c) Flow cytometric analysis of the expression of Ig isotypes and CD138 on iGB cells, and of Fas and GL7 on CD138−gated cells, cultured as in (a). Colours of the boxes indicate the culture conditions described in (a). Numbers indicate the percentages of cells in the quadrants or windows. Data shown are representative of five independent experiments. As shown in Figure 5b , proliferation was greater in the secondary culture with IL-21 than with IL-4, and the IgG1 + cells dominated over IgE + cells, which was opposite the case in the parallel IL-4 culture ( Fig. 5c ). We designated iGB cells cultured with IL-4 as iGB-4, and with IL-21 in the secondary culture as iGB-21 cells. The iGB-21 cells maintained logarithmic proliferation in further culture with IL-21 until day 8, expanding 10,000-fold ( Fig. 5b ). Whereas the frequency of CD138 + cells was increased only among the IgE + iGB-4 cells, it was increased in both IgE + and IgG1 + iGB-21 cells on day 8 ( Fig. 5c ), perhaps correlating with the preferential contribution of IL-4 and IL-21 to IgE and IgG1 antibody production, respectively, in TD immune responses [12] , [45] . Parallel culture of the iGB-21 cells on 40LB cells without cytokines from day 6 (iGB-m cells) resulted in a lower growth rate. The majority of the iGB-m cells as well as iGB-21 and iGB-4 cells were CD138 − and exhibited a GC phenotype (Fas + and GL7 + ) ( Fig. 5c ). These results indicate that IL-21 promotes extensive proliferation and partial differentiation towards PC of iGB cells in vitro . Figure 5: IL-21 accelerates proliferation of iGB cells and partial differentiation of IgG1 + iGB cells into plasmablasts. ( a ) Schematic diagram of the different iGB cell cultures performed in ( b , c ). In vitro generated iGB cells were successively cultured on 40LB cells with IL-4 (iGB-4; black), or with IL-21 replacing IL-4 on day 4 (iGB-21; red). Additionally, the iGB-21 cells were deprived of IL-21 on day 6 and successively cultured on 40LB without added cytokines (iGB-m; blue). ( b ) Cumulative fold increase on day 4, 6, and 8, of B cells cultured as described in ( a ) was estimated from three independent experiments and represented as in Figure 1b . Colours of the lines indicate the culture conditions described in ( a ). ( c ) Flow cytometric analysis of the expression of Ig isotypes and CD138 on iGB cells, and of Fas and GL7 on CD138 − gated cells, cultured as in ( a ). Colours of the boxes indicate the culture conditions described in ( a ). Numbers indicate the percentages of cells in the quadrants or windows. Data shown are representative of five independent experiments. Full size image Compared with the CD138 − iGB-4 cells, expression of Bcl-6 and Bcl-xL proteins was lower in the CD138 − iGB-21 cells, but higher than in ex vivo GC B cells ( Fig. 1g ). The messenger RNA levels of Aicda, which encodes activation-induced cytidine deaminase (AID) that is indispensable for CSR and SHM, was ∼ 4- or ∼ 10-fold lower in the IgG1 + iGB-4 or iGB-21 cells, respectively, than the GC B cells ( Supplementary Fig. S6 ). In relation to this diminished level of Aicda expression, the iGB-21 cells derived from B1-8 ki B cells had no detectable V H gene mutations on day 8 of the culture with or without continuous BCR stimulation by anti-κ antibody. Forced expression of AID in the iGB cells ( Supplementary Methods ) resulted in the accumulation of V H mutations. The mutation rate was estimated as 1.5×10 −4 per base pair per generation (roughly estimated as 8 generations after AID expression), which was within the range reported in physiological GC B cells [46] ( Supplementary Fig. S6 ). The mutations consisted of C-to-T/G-to-A transitions, possibly generated through AID-mediated C-deamination, as well as other substitutions and a deletion, typical of the mutations normally seen in immunized animals, suggesting that iGB cells possess all of the essential SHM machinery operative in physiological GC B cells [47] . This result also suggests that a higher level of AID is required for SHM than for CSR. IL-21 reversibly suppresses iMB cell development from iGB cells To examine the effect of IL-21 on the in vivo differentiation of iGB cells into iMB cells, we transferred an equal number of IgG1 + CD138 − Ly5.1 + , iGB-4, iGB-21 or iGB-m cells into C57BL/6 mice and analysed them 30 days later. Ly5.1 + iMB cells were detected in the spleen, lymph node, peritoneal cavity(PerC), and blood from the iGB-4 cell (iMB-4) and iGB-m cell (iMB-m) recipients ( Fig. 6a ). Most of the iMB cells were IgG1 + but never IgE + ( Supplementary Fig. S7 ). Absolute numbers of iMB-4 and iMB-m cells in the recipient spleens were 2–5×10 5 and 0.5–1×10 5 , respectively, 30–50 days after the transfer, and gradually decreased thereafter ( Fig. 6b ). In striking contrast, essentially no iMB cells were detected in the mice adoptively transferred with iGB-21 cells ( Fig. 6a,b ). 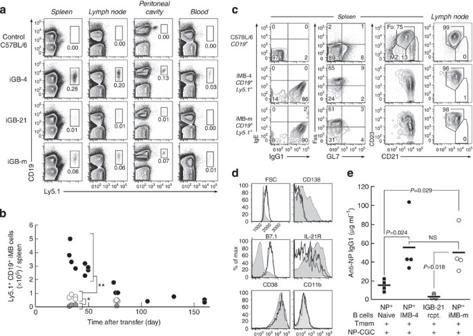Figure 6: IL-21 reversibly suppresses the differentiation of iGB cells into iMB cells. (a) Flow cytometric analysis for CD19/Ly5.1 expression on the cells from indicated tissues of untreated C57BL/6 mice (B6) or recipient mice that received iGB-4, iGB-21, or iGB-m cells, each devoid of CD138−cells and containing 1×107IgG1+cells, 30 days before. The numbers indicate the percentage of iMB cells defined by each window. (b) The numbers of splenic iMB-4 (closed circles:n=15), iMB-21 (shaded circles:n=4) or iMB-m (open circles:n=8) cells were estimated by the analysis as shown in (a) in individual recipient mice on the indicated days. Difference is significant between the iMB-4 and iMB-m cells (**P<0.000006) and between iMB-m and iMB-21 cells (*P<0.01) from the recipient mice analysed by day 50 after transfer. Data from 11 experiments were combined. (c) iMB-4 and iMB-m cells (CD19+Ly5.1+) in the spleens of mice generated as in (a) and in control CD19+B cells from untreated B6 mice were analysed for expression of the indicated markers. The numbers indicate the percentage of cells defined by each window. (d) Expression of the indicated markers on the splenic iMB-4 (thick line), iMB-m (dotted line) or B6 naïve (shaded) B cells. (c,d) Data shown are representative of three or more independent experiments. (e) Splenic B cells of the recipient mice containing 8×103NP+iMB-4 or iMB-m cells, or those of a B1-8 ki mouse containing 8×103NP+naïve B cells (the numbers were estimated on the basis of their frequency in flow cytometric analyses), each supplemented with naïve B cells of untreated B6 mice to make the total B-cell number 2.4×107, or splenic B cells (2.4×107) of the recipient having received iGB-21 cells ('iGB-21 rcpt.'), were co-transferred with CGG-primed CD4+T cells (Tmem) into γ-irradiated B6 mice. Seven days after i.v. immunization with NP40-CGG, serum titres of anti-NP IgG1 in individual mice (n=4 for each group) were measured. Data shown are representative from two independent experiments. Figure 6: IL-21 reversibly suppresses the differentiation of iGB cells into iMB cells. ( a ) Flow cytometric analysis for CD19/Ly5.1 expression on the cells from indicated tissues of untreated C57BL/6 mice (B6) or recipient mice that received iGB-4, iGB-21, or iGB-m cells, each devoid of CD138 − cells and containing 1×10 7 IgG1 + cells, 30 days before. The numbers indicate the percentage of iMB cells defined by each window. ( b ) The numbers of splenic iMB-4 (closed circles: n =15), iMB-21 (shaded circles: n =4) or iMB-m (open circles: n =8) cells were estimated by the analysis as shown in ( a ) in individual recipient mice on the indicated days. Difference is significant between the iMB-4 and iMB-m cells (** P <0.000006) and between iMB-m and iMB-21 cells (* P <0.01) from the recipient mice analysed by day 50 after transfer. Data from 11 experiments were combined. ( c ) iMB-4 and iMB-m cells (CD19 + Ly5.1 + ) in the spleens of mice generated as in ( a ) and in control CD19 + B cells from untreated B6 mice were analysed for expression of the indicated markers. The numbers indicate the percentage of cells defined by each window. ( d ) Expression of the indicated markers on the splenic iMB-4 (thick line), iMB-m (dotted line) or B6 naïve (shaded) B cells. ( c , d ) Data shown are representative of three or more independent experiments. ( e ) Splenic B cells of the recipient mice containing 8×10 3 NP + iMB-4 or iMB-m cells, or those of a B1-8 ki mouse containing 8×10 3 NP + naïve B cells (the numbers were estimated on the basis of their frequency in flow cytometric analyses), each supplemented with naïve B cells of untreated B6 mice to make the total B-cell number 2.4×10 7 , or splenic B cells (2.4×10 7 ) of the recipient having received iGB-21 cells ('iGB-21 rcpt. '), were co-transferred with CGG-primed CD4 + T cells (T mem ) into γ-irradiated B6 mice. Seven days after i.v. immunization with NP 40 -CGG, serum titres of anti-NP IgG1 in individual mice ( n =4 for each group) were measured. Data shown are representative from two independent experiments. Full size image The iMB-m cells had the same memory phenotype as iMB-4 cells ( Fig. 6c,d ; Supplementary Fig. S7 ). Both types of iMB cells in the spleen, but not in lymph node, exhibited a phenotype similar to MZ B cells in terms of CD21 versus CD23 expression ( Fig. 6c ), and expressed a low level of IL-21R, as reported for human B mem cells [48] ( Fig. 6d ; Supplementary Fig. S7 ). The iMB-m cells were comparable to iMB-4 cells in their function to respond to soluble Ag in the secondary recipient mice, whereas B cells from the iGB-21-recipients, which contain no discernable iMB cells, failed to respond ( Fig. 6e ). These results indicate that the ability of iGB cells to differentiate into functional iMB cells is inhibited by IL-21 in vitro , and also that this inhibition is reversible. IL-21 facilitates LLPC development from iGB cells LLPCs are generated during the late phase of the GC reaction [9] ; therefore, we examined whether iGB cells differentiate into LLPCs by estimating the number of Ab-forming cells (AFC) in the bone marrow (BM) of mice that received IgG1 + NP + CD138 − iGB cells derived from B1-8 ki mice. Anti-NP IgG1-secreting AFCs were detected in mice that received iGB-21 cells 4 weeks previously, but very few were seen in mice that received iGB-4 or iGB-m cells ( Fig. 7a ). Similarly, AFCs in spleen were only found in the mice receiving iGB-21 cells. The iGB-21-derived LLPCs were undetectable by flow cytometry, probably because of their scarcity ( ∼ 0.005% as estimated from the data in Fig. 7a ) and also because Ly5.1 (CD45.1) is downregulated on PCs [49] . Serum anti-NP IgG1 titres correlated with the AFC numbers in the different recipient mice. The IgG1 + CD138 − iGB-21 cells appeared to be committed to the plasma-cell lineage because Blimp1 mRNA expression level was relatively high in these cells, whereas it was very low in the IgG1 + CD138 − iGB-4 or iGB-m cells, each cultured for the same time period as the iGB-21 cells ( Fig. 7b ). Moreover, nearly 40% of the IgG1 + CD138 − iGB-21 cells on day 6, and even more on day 8, were secreting anti-NP IgG1, whereas essentially none of the IgG1 + CD138 − iGB-4 (on day 6) or iGB-m (on day 8) cells were secreting ( Fig. 7c ). These data indicate that secondary culture with IL-21 induces differentiation of iGB cells into CD138 − AFCs, presumably the early precursors of LLPCs, but the CD138 − AFCs disappear during the subsequent culture without IL-21. As expected, CD138 + iGB cells arising in any culture condition expressed high levels of Blimp1 mRNA and were mostly AFCs ( Fig. 7b,c ). 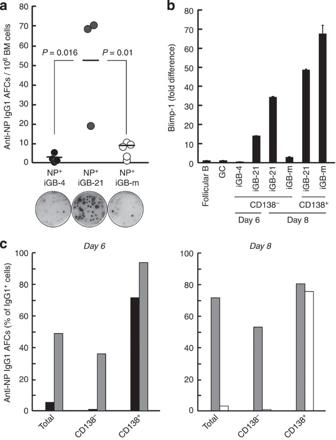Figure 7: IL-21 promotes differentiation of iGB cells towards plasma cells. (a) The frequency of NP-specific IgG1 AFCs among BM cells determined by ELISPOT assay. Shown is collective data with averages (bars) from five experiments using individual mice that had received iGB-4 (n=4), iGB-21 (n=3), or iGB-m (n=5) CD138−IgG1+NP+iGB cells derived from B1-8 ki mice 26–30 days before. Photographs depict representative ELISPOT wells seeded with 5×105total BM cells. (b) Quantitative real-time PCR analysis of Blimp-1 transcripts in the following cells: splenic follicular B cells (CD43−, CD138−, CD19+, CD23high, CD21+) sorted from unimmunized C57BL/6 mice, physiological GC B cells (CD43−, CD138−, IgD−, CD19+, Fas+, GL7+) sorted from C57BL/6 mice immunized with BSA/CFA 3 weeks before, CD138−IgG1+cells sorted from iGB-4, iGB-21 or iGB-m cells, and CD138+cells from iGB-21 or iGB-m cells, each collected on the indicated day of the culture. Expression levels relative to that in follicular B cells (set as 1) are shown. Data is representative of two independent experiments. Error bars represent s.d. of triplicate samples. (c) CD138+or CD138−and IgG1+cells were purified by MACS from iGB-4 and iGB-21 cells on day 6 or iGB-21 and iGB-m cells on day 8, and the frequency of anti-NP IgG1+AFCs in these cells and pre-purified total IgG1+cells was determined by ELISPOT. iGB-4, iGB-21 and iGB-m cells are shown as black, grey and white bars, respectively. Data is representative of two independent experiments. Figure 7: IL-21 promotes differentiation of iGB cells towards plasma cells. ( a ) The frequency of NP-specific IgG1 AFCs among BM cells determined by ELISPOT assay. Shown is collective data with averages (bars) from five experiments using individual mice that had received iGB-4 ( n =4), iGB-21 ( n =3), or iGB-m ( n =5) CD138 − IgG1 + NP + iGB cells derived from B1-8 ki mice 26–30 days before. Photographs depict representative ELISPOT wells seeded with 5×10 5 total BM cells. ( b ) Quantitative real-time PCR analysis of Blimp-1 transcripts in the following cells: splenic follicular B cells (CD43 − , CD138 − , CD19 + , CD23 high , CD21 + ) sorted from unimmunized C57BL/6 mice, physiological GC B cells (CD43 − , CD138 − , IgD − , CD19 + , Fas + , GL7 + ) sorted from C57BL/6 mice immunized with BSA/CFA 3 weeks before, CD138 − IgG1 + cells sorted from iGB-4, iGB-21 or iGB-m cells, and CD138 + cells from iGB-21 or iGB-m cells, each collected on the indicated day of the culture. Expression levels relative to that in follicular B cells (set as 1) are shown. Data is representative of two independent experiments. Error bars represent s.d. of triplicate samples. ( c ) CD138 + or CD138 − and IgG1 + cells were purified by MACS from iGB-4 and iGB-21 cells on day 6 or iGB-21 and iGB-m cells on day 8, and the frequency of anti-NP IgG1 + AFCs in these cells and pre-purified total IgG1 + cells was determined by ELISPOT. iGB-4, iGB-21 and iGB-m cells are shown as black, grey and white bars, respectively. Data is representative of two independent experiments. Full size image We have described a novel B-cell culture system in which naïve B cells proliferate robustly, undergo isotype switching, and acquire a cell surface phenotype equivalent to GC B cells, termed iGB cells. After primary culture with IL-4 (iGB-4 cells), the cells develop into memory-like iMB cells in vivo , whereas after subsequent culture with IL-21 (iGB-21 cells) develop into LLPC-like cells in vivo . Bcl-6 and Bcl-xL proteins, which are among the signature proteins of physiological GC B cells [38] , are abundantly expressed in iGB-4 and iGB-21 cells. It was recently reported that human peripheral memory B cells transduced with Bcl-6 and Bcl-xL could be propagated as GC-like B cells for a long period on feeder cells expressing CD40L and supplemented with IL-21 (ref. 50 ). Thus, the high-level expression of Bcl-6 and Bcl-xL, together with signalling through CD40 and the IL-21 receptor, seem to be required for the extensive B-cell proliferation in vitro . In our system, initiating the culture with IL-21 resulted in a poor proliferation of the iGB cells, suggesting that the primary IL-4-receptor signalling may be required for sufficient upregulation of Bcl-6 and Bcl-xL proteins in naïve B cells. Somewhat unexpectedly, the level of Bcl-6 mRNA was low in iGB cells compared with ex vivo GC B cells ( Supplementary Figs S6 and S8 ). However, it is well known that Bcl-6 mRNA and protein levels can be discordant. For example, resting and GC B cells have similar Bcl-6 message levels, yet Bcl-6 protein levels are much higher in the GC B cells, suggesting an important role for post-transcriptional regulatory mechanisms [51] . CD40 signalling has been shown to suppress Bcl-6 transcription via Irf4 (refs 51 , 52 ). As both iGB-4 and iGB-21 cells express abundant Irf4 protein ( Fig. 1g ), the continuous stimulation through CD40 in the culture may cause the suppression of Bcl-6 gene expression. Thus, Bcl-6 protein must be induced in the initial phase of the primary culture with IL-4 and maintained with only slow decay during the secondary culture with IL-21 ( Fig. 1g ). The levels of Bcl-6 protein may reach an insufficient level around day 10, when the iGB-21 cells stop proliferating. This assumption is supported by our preliminary data demonstrating that retroviral transduction of Bcl-6 endowed the iGB-21 cells with unlimited growth capacity in the presence of IL-21 and 40LB feeder cells. Despite their GC-like phenotype and high proliferative potency, the iGB-21 cells failed to mutate their Ig genes, a feature at least partly due to insufficient expression of AID for unknown reasons. The decreasing level of AID mRNA expression in iGB-21 cells inversely correlated with the increasing level of Blimp-1 mRNA ( Supplementary Fig. S6 and Fig. 7b ), and therefore Blimp-1 might downregulate the AID gene expression as proposed previously [53] . One prominent feature of this system is that the developmental fate of the iGB cells, either becoming B mem cells or LLPCs, can be directed by cytokines. IL-4 directs the cells to the iMB cell fate, but not into LLPCs, in vivo . The iMB cells exhibit a uniform B mem phenotype, persist in vivo for months without cell division, and rapidly differentiate into PCs in the red pulp of the spleen in response to soluble TD antigen. These features confirm that the iMB cells are physiologically equivalent to B mem cells. Given this premise, it is noteworthy that iMB cells are induced in vitro and develop in vivo in the absence of antigenic stimulation through the BCR. This indicates that, apart from its function for Ag presentation to T cells, BCR signalling per se is not necessary for GC B cells to become B mem cells, in agreement with studies showing a sufficient memory recall response in Btk- and BLNK-deficient mice [54] , [55] . It is also an intriguing finding that no specific GC microenvironment is required for B mem cell development, because the recipient mice do not develop GC. This result is consistent with previous findings that premature B mem cells can be produced in mice in which germinal centre formation is inhibited by anti-ICOS Ab administration [56] or Bcl-6 deficiency [27] . IgM/D + iMB cells possessing all the same features as IgG1 + iMB cells, except for the Ig isotype, are generated at the same time as IgG1 + iMB cells, and they may correspond to the IgM + B mem cells first identified in the TD immune response of Bcl-6-deficient mice [27] . In contrast, IgE + iMB cells are not generated in vivo from IgE + iGB cells. Expression levels of BAFF-R, a receptor for a B-cell survival factor, cannot account for this deficiency, because they were almost equal between IgE + and IgG1 + iGB-4 cells ( Supplementary Fig. S1 ). It seems more likely that IgE + iGB-4 cells are committed to differentiation towards PCs, as Blimp-1 mRNA levels were tenfold higher in the IgE + iGB-4 cells than in the IgG1 + iGB-4 cells, among other GC-related mRNAs, although still much lower than in PCs ( Supplementary Fig. S8 ). This idea is consistent with the fact that IgE + cells arising from IgG + GC B cells swiftly become PCs and that IgE + B mem cells are barely detectable in mice even after immunization to induce an optimal IgE response [5] . B-cell intrinsic IL-21 signalling is necessary for optimal GC formation and high-affinity IgG1-producing LLPC formation during TD immune responses [9] , [10] , [11] , [12] . Accordingly, we demonstrated here that IL-21 maintained the logarithmic proliferation of iGB cells after primary culture with IL-4 and that the CD138 − fraction of the iGB-21 cells differentiated to LLPCs, but not to iMB cells, in vivo . Perhaps relevant to this observation, Tarlinton and colleagues reported accelerated formation of B mem cells that had undergone less SHM and affinity maturation in IL-21- or IL-21R-deficient mice, suggesting premature development of B mem cells in the GC reaction [9] . Collectively, these observations suggest that IL-21 normally suppresses the differentiation of GC B cells towards B mem cells and instead promotes their differentiation towards LLPCs. Notably, this suppression was reversible in at least a fraction of iGB cells, allowing iMB cell development from the iGB cells after IL-21 deprivation (iGB-m cells). This reversible suppression did not directly correlate to the expression level of BAFF-R on the iGB cells ( Supplementary Fig. S1 ), although the evaluation of surface BAFF-R here might have been compromised owing to possible downregulation by continuous stimulation with BAFF produced from the feeder cells in the prolonged culture. Whatever the mechanism for the IL-21-mediated suppression, this finding suggests that the iGB cells maintain plasticity in their differentiation potential for at least a few days under IL-21 stimulation. If this were to apply to a physiological GC B cell reaction, IL-21 might afford GC B cells sufficient time to be diversified and selected before their fate is determined. After this period, positively selected GC B cells would differentiate into either LLPC or B mem cells, depending on further availability of IL-21. Preparation of feeder cells Mouse CD40L complementary DNA cloned into a pApuro2 expression vector (a gift of Dr T. Kurosaki) was transfected into BALB/c3T3 fibroblasts (clone A31, provided by RIKEN BRC) by lipofection and puromycin (5 μg ml −1 )-resistant stable clones (40L cells) were subsequently selected. Mouse BAFF cDNA cloned into a pCA-neo, a T7-tag-deleted variant of the pCAT7-neo expression vector [57] , was transfected into the 40L or 3T3 cells and G418 (2 mg ml −1 )-resistant clones were subsequently selected. Among the 40L transfectants, a clone on which naïve B cells proliferated most extensively in the presence of IL-4 was named 40LB and used for the rest of the experiments. All BALB/c3T3-derived cells were mycoplasma-free as determined using the PCR Mycoplasma Detection Set (Takara). Mice C57BL/6 mice were purchased from Japan SLC. B1-8 IgH knock-in (B1-8 ki) mice [42] were backcrossed to C57BL/6 or congenic C57BL/6-Ly5.1 strains. Hy10 (formerly called HyHEL10) mice carrying a V H knock-in (VDJ9 ki) allele and an Ig-κ transgene (κ5 tg) [40] , [41] were backcrossed to C57BL/6 or the congenic C57BL/6-Ly5.1 strains. All mice were maintained in the mouse facility under specific pathogen-free conditions. Mouse procedures were performed under protocols approved by the Animal Care and Use Committee of the Tokyo University of Science. Isolation of cells Single-cell suspensions from lymphoid tissues were depleted of RBCs in ammonium chloride lysis buffer and then incubated with 2.4G2 (BD Biosciences) to block FcγRII/III before staining with other Abs. Naïve B cells were purified from the spleens by 2-step negative sorting, first by an iMag system (BD Biosciences) using biotinylated monoclonal Abs (mAbs) against CD43 (BD Biosciences), CD4, CD8, DX5, Ter-119 (eBioscience), and avidin-particle-DM (BD Biosciences) and then by passing of the unbound cells through a MACS LS column (Miltenyi Biotec), yielding B cells of >97% purity. NP + B cells were enriched from the purified splenic B cells of B1-8 ki mice with a MACS system using NP 7 -BSA-biotin, yielding NP + cells of >50% purity. About 50% of purified B cells from Hy10 Ly5.1 + mice were HEL-binding and used without further purification. Follicular and MZ B cells from Hy10 mice were sorted by FACSAria II (BD Biosciences) after staining with CD21-FITC, CD23-PE (BioLegend), and CD19-allophycocyanin(APC) (eBioscience). CD4 + T cells from mice immunized with alum-precipitated CGG were purified with an iMag system using biotinylated mAbs against CD45R/B220, CD8, and CD11b (eBioscience), yielding CD4 + T cells of >70% purity. For removal of feeder and plasmablasts/plasma cells, single-cell suspensions from the iGB cultures were first incubated with 2.4G2 and then with biotinylated mAbs against H-2Kd and CD138 (BD Biosciences) at room temperature in MACS Buffer (0.5% BSA, 2 mM EDTA in PBS), followed by incubation with avidin-particle-DM (BD Biosciences) and purification by an iMag system. Thus purified iGB cells were used for the adoptive transfer into irradiated recipient mice. iGB cell culture Typically, purified B cells (5×10 5 cells per dish) were cultured in a 10-cm tissue culture dish (BD Falcon) in the presence of 40LB cells (3×10 6 cells per dish) that had been irradiated with 120 Gy γ-ray in 40 ml RPMI-1640 medium (Sigma) supplemented with 10% FCS, 5.5×10 −5 M 2-ME, 10 mM HEPES, 1 mM sodium pyruvate, 100 units ml −1 penicillin, and 100 μg ml −1 streptomycin (GIBCO). rIL-4 (1 ng ml −1 ; Peprotech) was added to the primary culture for 4 days, and on day 4, the cells were re-plated onto a new feeder layer and cultured with rIL-21 (10 ng ml −1 ; Peprotech) or IL-4 for 2–4 days (the secondary culture). In tertiary culture, cells were cultured on a new feeder layer without extra cytokines. Each time the cells were collected, the live B cell number was counted by the trypan blue dye exclusion method. Cells were cultured in a humidified atmosphere at 37 °C with 5% CO 2 . Flow cytometry Cells from lymphoid tissues depleted of RBCs were incubated with 2.4G2 and then stained with various combinations of the following Abs: FITC-, PE-, biotin-, PE-Cy7-, or APC-conjugated anti-mouse IgD, IgM, IgG1, and IgE (Southern Biotechnology), anti-mouse CD45.1 (BioLegend), anti-mouse CD5, CD19, CD21, CD23, CD38, CD40, CD45R/B220, CD80, CD138, CD154, CD11b, MHC-class II, PNA, and GL7 (eBioscience), anti-mouse CD43 (S7), CD95 (BD Biosciences), biotinylated-HEL, and biotinylated NP 7 -BSA. The concentrations of the Abs used in this study are shown in the Supplementary Table S1 . IL-21R was detected by a mouse IL-21–human Cγ1 fusion protein combined with PE-goat-anti-human IgG. Cells were stained with propidium iodide, just before analysis, to eliminate dead cells in the data analyses. When the iGB cells were analysed, 40LB feeder cells were gated out based on FSC versus SSC. CFSE labelling was performed according to the manufacturer's instructions (Molecular Probes) in that freshly isolated splenic B cells (1×10 7 cells per ml) were incubated with 2.5 μM CFSE in 0.05% BSA in PBS at 37 °C for 10 min and then stained as above and used for the experiments. All samples were analysed using a FACSCalibur or FACSCanto II (BD Biosciences). The data were analysed using FlowJo (Tree Star). BrdU labelling and detection B cells were pulsed with 10 μM BrdU for the last 1 h on day 3 or 7 h on day 4 of iGB culture. Single-cell suspensions were stained for surface markers as described above, washed with cold PBS, and resuspended in 0.5 ml of cold 0.15 M NaCl, to which 1.2 ml of cold 95% ethanol was added dropwise while the tube was weakly vortexed and kept 30 min on ice. Cells were washed and fixed with 1 ml of 1% paraformaldehyde/PBS containing 0.05% Tween 20 overnight at 4 °C. Fixed cells were resuspended in 1 ml of 0.15 M NaCl, 4.2 mM MgCl 2 , and 10 μM HCl containing 30 U ml −1 DNase I (Sigma-Aldrich) and then incubated for 30 min at room temperature. After being washed twice with PBS, cells were stained overnight at 4 °C with FITC-conjugated anti-BrdU (BD Biosciences) and analysed with FACSCanto II. Western blot analysis Cell samples were lysed in 1× SDS–PAGE sample buffer, sonicated, boiled and used for SDS–PAGE followed by Western blotting. The following primary polyclonal antibodies were used: rabbit anti-Bcl-6 (Cell Signaling), rabbit anti-BcL-xL (S-18), goat anti-Irf4 (M-17) and rabbit anti-Syk (N-19) (Santa Cruz Biotechnology), and rabbit β-actin (Abcam). Goat anti-rabbit IgG-HRP and rabbit anti-goat IgG-HRP (Zymed) were used as secondary antibodies. ECL western blotting detection reagents (Amersham) were used for detection. Immunization and adoptive transfer Purified iGB cells (2×10 7 ) derived from Hy10 or B1-8ki mice of C57BL/6-Ly5.1 background were injected i.v. into γ-irradiated (6.5 Gy) C57BL/6 mice (Ly5.2 + ). After ≥30 days, B cells purified from pooled spleens of the recipient mice were analysed by flow cytometry, as described above, and HEL- or NP-specific iMB cells, defined as CD19 + Ly5.1 + , were enumerated. To examine the immune response of these iMB cells, whole spleen cells from the mice previously immunized with OVA/complete Freund's adjuvant (CFA) or CD4 + T cells from those immunized with CGG/alum, both including memory T cells, were mixed with splenic B cells containing equal number of iMB cells and transferred into C57BL/6 mice. Twelve hours later, recipients were immunized i.v. with OVA-HEL (20 μg) or NP 40 -CGG (25 μg) in PBS and bled from the tail vein for ELISA on the indicated days after immunization. ELISA and ELISPOT assays NP-specific AFCs in BM or purified iGB cells were detected using an ELISPOT assay on a MultiScreen 96-well filtration plate (Millipore) coated with 10 μg ml −1 NP 9 -BSA. Serially diluted cells were added to individual wells in triplicate and then incubated for 6 h in a humidified atmosphere at 37 °C with 5% CO 2 . Anti-NP IgG1 spots were revealed by HRP-conjugated goat anti-mouse IgG1 Ab (Southern Biotechnology) in conjunction with AEC substrate (DAKO). ELISA was performed as follows: flat-bottom 96-well plates (NUNC) were coated with NP 9 -BSA (10 μg ml −1 ) or HEL (2 μg ml −1 ; Sigma) and blocked with 10% FCS or 3% BSA in PBS, respectively, and serially diluted serum samples were then added to individual wells. Bound Abs were revealed by HRP-conjugated goat anti-mouse IgG1 Ab (Southern Biotechnology) in conjunction with TMB substrate (Sigma). Absorbance at 450 nm was measured using a Benchmark microplate reader (Bio-Rad). mAbs binding with high affinity to HEL (C2) [58] or NP (C6) [59] , respectively, were used as standards. Immunofluorescence microscopy Immunized spleens were embedded in O.C.T. compound (Sakura), frozen in liquid nitrogen, and stored at −80 °C. Frozen sections (7 μm thick) were fixed in −20 °C acetone for 15 s. After being washed with a buffer (0.01% Tween 20 in PBS), the sections were pre-incubated with a staining buffer (0.01% Tween 20 and 3% BSA in PBS) containing 2.4G2 (1 μg ml −1 ) for 30 min at room temperature. The sections were stained with 0.7 μg ml −1 biotinylated HEL (HEL-biotin), 5 μg ml −1 anti-B220-APC (eBioscience), Alexa-647-conjugated anti-MAdCAM1, anti-Thy1.2-FITC, anti-B220-FITC (BD Biosciences) and/or goat anti-IgG1-FITC (Southern Biotechnology) as indicated followed by PE-conjugated avidin (1 μg ml −1 ; eBioscience). After washing, the slides were mounted with Fluorescent Mounting medium (Dako). The samples were examined by immunofluorescence microscopy (BZ-9000; Keyence). Quantitative RT–PCR RNA from sorted B cells was prepared with RNeasy (Qiagen). The ReverTra Ace first-strand cDNA synthesis kit (Toyobo) was used to prepare cDNA. Quantitative real-time PCR was performed with the Power SYBR Green PCR Master Mix (Applied Biosystems) and a 7500 Fast Real-Time PCR System (Applied Biosystems) according to standard PCR conditions. Gene expression was normalized to that of Gapdh (encoding glyceraldehyde-3-phosphate dehydrogenase) and data are presented as a fold difference of the normalized values relative to that of follicular B cells by the '2-ΔΔCT' (change in cycling threshold) method. The following primer sets were used: Gapdh sense: 5′-ggagaaacctgccaagtatga-3′; Gapdh antisense: 5′-ccctgttgctgtagccgtatt-3′; Blimp-1 sense: 5′-gaacctgcttttcaagtatgctg-3′; Blimp-1 antisense: 5′-agtgtagacttcaccgatgagg-3′. Statistical analysis Statistical analysis was performed using the Student's t -test. How to cite this article: Nojima, T. et al . In-vitro derived germinal centre B cells differentially generate memory B or plasma cells in vivo . Nat. Commun. 2:465 doi: 10.1038/ncomms1475 (2011).